Staged decline of neuronal functionin vivoin an animal model of Alzheimer's disease The accumulation of amyloid-β in the brain is an essential feature of Alzheimer's disease. However, the impact of amyloid-β-accumulation on neuronal dysfunction on the single cell level in vivo is poorly understood. Here we investigate the progression of amyloid-β load in relation to neuronal dysfunction in the visual system of the APP23×PS45 mouse model of Alzheimer's disease. Using in vivo two-photon calcium imaging in the visual cortex, we demonstrate that a progressive deterioration of neuronal tuning for the orientation of visual stimuli occurs in parallel with the age-dependent increase of the amyloid-β load. Importantly, we find this deterioration only in neurons that are hyperactive during spontaneous activity. This impairment of visual cortical circuit function also correlates with pronounced deficits in visual-pattern discrimination. Together, our results identify distinct stages of decline in sensory cortical performance in vivo as a function of the increased amyloid-β-load. While learning and memory defects are key symptoms of Alzheimer's disease (AD) [1] , patients progressively exhibit complex cognitive impairments [2] , and even deficits in central sensory processing, particularly at advanced stages of their disease. Thus, different sensory modalities can be affected [3] , [4] , [5] including information processing in the visual system [6] , [7] , [8] , [9] . The amyloid-β (Aβ)-peptide has been identified as a key molecule in the pathogenesis of AD. It accumulates in various forms in AD brains, including soluble oligomeric entities and insoluble Aβ-plaques [10] . The presence of Aβ-plaques is a defining criterion for the diagnosis of AD [1] . In vitro studies have suggested different mechanisms of action for Aβ, including changes in ion-channel properties [11] , [12] , [13] , impairments of synaptic transmission and synaptic plasticity of individual neurons exposed to Aβ [14] , [15] , [16] , [17] , [18] . In addition, morphological studies have revealed abnormal geometries of dendrites and axons in post-mortem human brains of AD patients [19] as well as neuritic dystrophies and a loss of dendritic spines in brains of AD mouse models [12] , [20] , [21] , [22] . These structural changes suggest that the accumulation of Aβ could lead to an impairment of neuronal signal integration and affect neuronal circuit function [19] , [22] . Effects of Aβ on the network level have also recently been investigated in vivo in different mouse models of AD [23] . Recordings of electrically evoked activity showed that synaptic integration is disrupted in the Aβ-plaques-containing cortex [22] . In addition, generalized spontaneous aberrant excitatory activity was recorded by electroencephalography in the cortex and the hippocampus of another AD mouse model [24] . Furthermore, local field potential recordings of oscillatory activity in the olfactory bulb and the piriform cortex revealed abnormal spontaneous and odour-related activity in the Tg2576 mouse model of AD [25] . Using two-photon calcium imaging, a recent study of the spontaneous ongoing activity in the frontal cortex identified two fractions of neurons with impaired activity [26] . In addition to a pronounced silencing of activity in a fraction of neurons, a separate fraction of neurons was found to be hyperactive in the Aβ-containing cortex. It remains an open question, however, how Aβ impacts the functionality of individual cortical neurons in vivo and how this is associated with a behavioural phenotype. Here we used the visual system of the APP23×PS45 mice as a cortical circuit model to investigate the relation between Aβ-load, neuronal circuit function and behavioural performance. The visual cortex is in many ways a well-suited model system for such a study, as neuronal networks underlying spontaneous and sensory-evoked activity can be examined in vivo . Thus, in the visual cortex, the functionality of a neuron within the cortical circuit can be directly evaluated in an anaesthetized animal by using specific visual stimuli. For example, one functional property of the visual neurons that can be directly assessed is their orientation selectivity, that is, their capacity to respond more significantly to one principal orientation of a visual stimulus than any other. To study neuronal network activity in the visual cortex in vivo , powerful experimental techniques are readily implemented in mouse models. In recent years, two-photon calcium imaging of cortical circuits allowed the simultaneous recording of the activity of multiple neurons in vivo , with single-cell resolution [27] , [28] , [29] , [30] . Furthermore, two-photon microscopy is increasingly used for the imaging of Aβ-related pathologies [20] , [21] , [31] . In the present study, we used in vivo two-photon calcium imaging to investigate the network effects of Aβ at the level of single cortical neurons in the APP23×PS45 transgenic mouse model of AD [32] , [33] . We imaged in vivo both the spontaneous and stimulus-evoked activity of neurons in the primary visual cortex of transgenic mice at different stages of the disease as well as of wild-type (WT) control mice. We also determined the Aβ-load, including both soluble Aβ and insoluble Aβ-plaques, of the visual cortex and the visual performance of the transgenic mice at different ages. Our results provide experimental evidence for the relation between cortical Aβ-load and functional impairments of neuronal circuits at the single cell level in vivo . Impaired tuning of visual cortex neurons in APP23×PS45 mice We assessed the functional properties of the visual cortex neurons by determining their orientation selectivity, that is, their capacity to respond better to one principal orientation of a visual stimulus than any other. The analysis of the neuronal tuning properties by in vivo two-photon calcium imaging allows the simultaneous analysis of the activity of many neurons in defined cortical layers [29] , [34] . These analyses rely on the recording of calcium transients in the neuronal cell bodies. It has been shown that these calcium transients directly reflect action potential firing (for example, refs 27 , 29 , 35 ). Here we examined neuronal calcium signals evoked by drifting grating stimulation in the primary visual cortex of aged (8–10 months) WT and APP23×PS45 mice. Drifting gratings were presented to the contralateral eye, while performing two-photon calcium imaging of neurons in the monocular region of the primary visual cortex after staining the tissue with the fluorescent calcium indicator dye OGB1-AM ( Fig. 1a ) [27] . 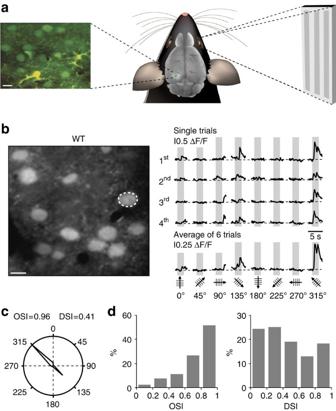Figure 1: Orientation and direction tuning of visual cortex neurons in 8–10 month-old WT mice. (a) Experimental arrangement forin vivotwo-photon calcium imaging of stimulation-evoked neuronal activity. Left panel,in vivotwo-photon image of cortical layer 2/3 of the primary visual cortex stainedin vivowith the fluorescent calcium indicator dye Oregon Green BAPTA-1 (green) and the glial marker Sulforhodamine 101 (yellow). Right panel, visual stimuli (drifting gratings) were projected on a screen placed 30 cm away from the contralateral eye of the mouse. (b) Left panel,in vivotwo-photon image of layer 2/3 neurons in the visual cortex of a WT mouse (8-months). Right panel, stimulus-evoked calcium transients recorded from the orientation selective neuron indicated in the left panel by a white dotted circle. Grey regions indicate periods of visual stimulation with drifting gratings schematized by oriented arrows on the bottom of each panel. Four single trials are represented on top and the average of six trials is shown below. Scale bar, 10 μm. (c) Polar plot showing the neuron's response function to oriented drifting gratings. The responses to each of the eight directions tested were normalized with respect to the maximal response. Then, the function was constructed by connecting the eight values. (d) Distribution of the orientation (OSI) and direction (DSI) selectivity indices of all responsive neurons (n=131 neurons) recorded in the visual cortices of 13 WT mice. Figure 1b illustrates an experiment that was performed in an 8-month-old WT mouse. In the field of view, we identified a neuron that showed large calcium transients for a specific orientation of the drifting gratings (directions of 135 and 315°), but no significant responses for all the other directions. A quantitative analysis of the stimulus-evoked responses showed that the neuron had an orientation selectivity index (OSI) of 0.96 and a direction selectivity index (DSI) of 0.41 (see also polar plot in Fig. 1c ). Thus, this neuron was defined as a highly tuned orientation-selective neuron [36] . On the whole, neurons from aged WT mice were found to be as highly tuned for orientation ( Fig. 1d ) as those in younger rodents [30] . Figure 1: Orientation and direction tuning of visual cortex neurons in 8–10 month-old WT mice. ( a ) Experimental arrangement for in vivo two-photon calcium imaging of stimulation-evoked neuronal activity. Left panel, in vivo two-photon image of cortical layer 2/3 of the primary visual cortex stained in vivo with the fluorescent calcium indicator dye Oregon Green BAPTA-1 (green) and the glial marker Sulforhodamine 101 (yellow). Right panel, visual stimuli (drifting gratings) were projected on a screen placed 30 cm away from the contralateral eye of the mouse. ( b ) Left panel, in vivo two-photon image of layer 2/3 neurons in the visual cortex of a WT mouse (8-months). Right panel, stimulus-evoked calcium transients recorded from the orientation selective neuron indicated in the left panel by a white dotted circle. Grey regions indicate periods of visual stimulation with drifting gratings schematized by oriented arrows on the bottom of each panel. Four single trials are represented on top and the average of six trials is shown below. Scale bar, 10 μm. ( c ) Polar plot showing the neuron's response function to oriented drifting gratings. The responses to each of the eight directions tested were normalized with respect to the maximal response. Then, the function was constructed by connecting the eight values. ( d ) Distribution of the orientation (OSI) and direction (DSI) selectivity indices of all responsive neurons ( n =131 neurons) recorded in the visual cortices of 13 WT mice. Full size image Next, we used the same approach to analyse aged APP23×PS45 mice ( Fig. 2 ). A remarkable feature of the visual cortex of these 8–10-month-old transgenic mice was the presence of Aβ-plaques ( Fig. 2a,b ) as well as a high amount of soluble Aβ (see below). We then studied the tuning properties of neurons in such Aβ-containing visual cortices. While some neurons had normal tuning properties, there was an increased incidence of neurons that were remarkably poorly tuned. For example, Fig. 2b illustrates the results obtained from such a neuron that happened to be located near an Aβ-plaque. Unlike the typical highly tuned neurons of WT mice, this neuron produced large calcium transients in response to several directions of the drifting grating stimulation. This relatively low level of tuning was reflected by the values for OSI (0.56) and DSI (0.22) (see also, polar plot in Fig. 2c ). A systematic analysis of the OSI and DSI in all recorded responsive neurons established the significantly reduced tuning performance of visual cortex neurons in aged APP23×PS45 mice ( Fig. 2d,e , Mann–Whitney test, OSI P <0.001, DSI P <0.05). 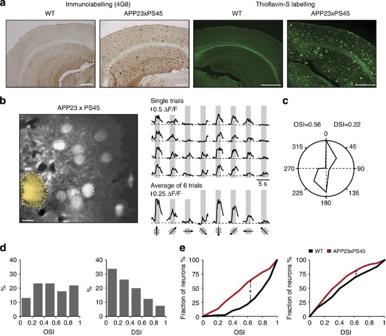Figure 2: Impaired orientation/direction tuning of visual cortex neurons in 8–10-month-old APP23×PS45 mice. (a) Amyloid-β-deposition in APP23×PS45 mice. Micrographs of coronal brain slices of visual cortices stained with the 4G8 antibody (a) and Thioflavin-S (b). The slices were obtained from a wild-type (WT, left panels) and an APP23×PS45 mouse (right panels) of the same age (9-months). Scale bars, 500 μm. (b) Left panel,in vivotwo-photon image of layer 2/3 neurons in the visual cortex of an APP23×PS45 mouse (8-months). The broken yellow line delineates a Thioflavin-S-positive plaque observed in the imaged focal plane. Right panel, stimulus-evoked calcium transients recorded from the neuron indicated by a white-dotted circle in the left panel. Grey regions indicate periods of visual stimulation with drifting gratings schematized by oriented arrows on the bottom of each panel. Single trials are represented on top and, the average of six trials is shown below. Scale bar, 10 μm. (c) Polar plot showing the neuron's response function to oriented drifting gratings. The responses to each of the eight directions tested were normalized with respect to the maximal response. Then, the function was constructed by connecting the eight values. (d) Distribution of the orientation (OSI) and direction (DSI) selectivity indices of all responsive neurons (n=145 neurons) recorded in the visual cortices of 15 APP23×PS45 mice. (e) Cumulative distributions of the orientation (OSI) and direction (DSI) selectivity indices determined for all responsive neurons recorded in WT (black) and APP23×PS45 (red) mice. Overall the visual cortex neurons of APP23×PS45 mice have significantly lower orientation and direction selectivities compared with WT ones (Mann–Whitney test, OSI, *P<0.001; DSI, *P<0.05). Figure 2: Impaired orientation/direction tuning of visual cortex neurons in 8–10-month-old APP23×PS45 mice. ( a ) Amyloid-β-deposition in APP23×PS45 mice. Micrographs of coronal brain slices of visual cortices stained with the 4G8 antibody ( a ) and Thioflavin-S ( b ). The slices were obtained from a wild-type (WT, left panels) and an APP23×PS45 mouse (right panels) of the same age (9-months). Scale bars, 500 μm. ( b ) Left panel, in vivo two-photon image of layer 2/3 neurons in the visual cortex of an APP23×PS45 mouse (8-months). The broken yellow line delineates a Thioflavin-S-positive plaque observed in the imaged focal plane. Right panel, stimulus-evoked calcium transients recorded from the neuron indicated by a white-dotted circle in the left panel. Grey regions indicate periods of visual stimulation with drifting gratings schematized by oriented arrows on the bottom of each panel. Single trials are represented on top and, the average of six trials is shown below. Scale bar, 10 μm. ( c ) Polar plot showing the neuron's response function to oriented drifting gratings. The responses to each of the eight directions tested were normalized with respect to the maximal response. Then, the function was constructed by connecting the eight values. ( d ) Distribution of the orientation (OSI) and direction (DSI) selectivity indices of all responsive neurons ( n =145 neurons) recorded in the visual cortices of 15 APP23×PS45 mice. ( e ) Cumulative distributions of the orientation (OSI) and direction (DSI) selectivity indices determined for all responsive neurons recorded in WT (black) and APP23×PS45 (red) mice. Overall the visual cortex neurons of APP23×PS45 mice have significantly lower orientation and direction selectivities compared with WT ones (Mann–Whitney test, OSI, * P <0.001; DSI, * P <0.05). Full size image Age-related increase in Aβ-load and impaired neuronal function To determine the relation between Aβ-load and cortical dysfunction, we examined three extra age groups at earlier stages of the disease (1.5–2, 3–3.25 and 4–4.5-month-old animals, Fig. 3 ). 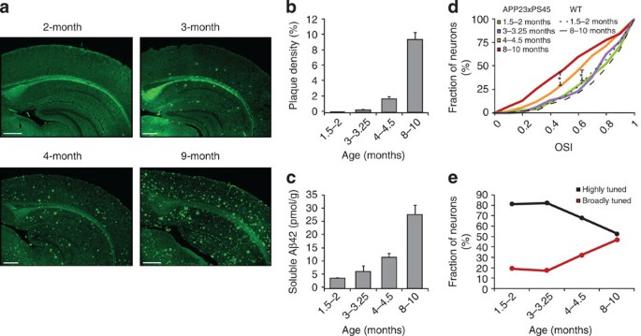Figure 3: Age dependence of amyloid-β-load and orientation tuning in the visual cortex of APP23×PS45 mice. (a) Amyloid-β-deposition in the visual cortex of APP23×PS45 mice. Micrographs of coronal brain slices of visual cortices stained with Thioflavin-S. The slices were obtained from 2-, 3-, 4- and 9-month-old APP23×PS45 mice. Scale bars, 500 μm. (b) Plaque density in the visual cortex of APP23×PS45 mice, determined in the four different age groups (1.5–2-, 3–3.25-, 4–4.5- and 8–10-month-old,n=5, 4, 5 and 6 mice, respectively). (c) Concentration of soluble Aβ42 in the forebrain of APP23×PS45 mice (n=5, 5, 6 and 5 mice, respectively). (d) Cumulative distributions of the OSIs determined for all responsive neurons recorded in APP23×PS45 mice at the different age groups (n=95, 94, 149 and 145 neurons in 7, 6, 8 and 15 mice, respectively) as well as in 1.5–2-month-old and 8–10-month-old WT mice (n=132 and 131 neurons in 7 and 13 mice, respectively). Functional impairments were observed only from the age of 4–4.5-months (Mann–Whitney test, APP23×PS45, 2-4-months, *P<0.005; 4–8-months, *P<0.005). (e) Proportion of highly (OSI>0.5) and broadly (OSI<0.5) tuned neurons in the visual cortex of APP23×PS45 mice (same neurons as ind). Figure 3a shows that plaques were absent at the age of 2 months, were sparse and present only in deeper layers in the cortex of 3-month-old mice, spread out also to upper cortical layers at the age of 4 months and, finally, were abundant and widely distributed in 9-month-old mice. A quantification of the age-dependent increase in plaque density, in the primary visual cortex, is provided in Fig. 3b . Although a similar development of plaques was observed in the lateral geniculate nucleus, no plaques were found in the retina throughout all ages tested in APP23×PS45 mice ( Supplementary Fig. S1 ). In addition, in the primary visual cortex, we found that the level of soluble Aβ paralleled the age-dependent increase in plaque density, although significant levels were already detected in the two youngest age groups ( Fig. 3c ). We then determined the tuning levels of visual cortex neurons in the four different age groups ( Fig. 3d,e ). Interestingly, the two earliest age groups studied, virtually lacking plaques, did not have measurable impairments in orientation selectivity ( Fig. 3d, e ). No significant difference was found between 1.5–2-month-old WT and APP23×PS45 mice ( Fig. 3d ; Mann–Whitney test, P =0.61) as well as between 1.5–2-month-old and 3–3.25-month-old APP23×PS45 mice ( Fig. 3d ; Mann–Whitney test, P =0.63). At the two later stages (4–4.5 and 8–10month), orientation tuning gradually decreased, as indicated by the upward shift of the cumulative distribution curves ( Fig. 3d ) and the relative changes of highly and broadly tuned neurons, respectively ( Fig. 3e ). Thus, during the first three months, neuronal orientation tuning was found to be normal and Aβ-plaques almost absent while soluble Aβ-levels were moderately increased. After the age of 4 months, the increase of Aβ-load, including both Aβ-plaques and soluble Aβ, was associated with the progressive impairment of orientation tuning of visual cortex neurons. To exclude the possibility that the PS45 mutation had an effect on neuronal tuning properties, we performed experiments in PS45 mice of 8–10 months of age. We found no significant difference in OSI or DSI between WT and PS45 mice ( Supplementary Fig. S2 ; Mann–Whitney test, OSI P =0.60, DSI P =0.23), indicating that the PS45 mutation alone is not sufficient for causing the neuronal deficits observed in APP23×PS45 mice. Figure 3: Age dependence of amyloid-β-load and orientation tuning in the visual cortex of APP23×PS45 mice. ( a ) Amyloid-β-deposition in the visual cortex of APP23×PS45 mice. Micrographs of coronal brain slices of visual cortices stained with Thioflavin-S. The slices were obtained from 2-, 3-, 4- and 9-month-old APP23×PS45 mice. Scale bars, 500 μm. ( b ) Plaque density in the visual cortex of APP23×PS45 mice, determined in the four different age groups (1.5–2-, 3–3.25-, 4–4.5- and 8–10-month-old, n =5, 4, 5 and 6 mice, respectively). ( c ) Concentration of soluble Aβ42 in the forebrain of APP23×PS45 mice ( n =5, 5, 6 and 5 mice, respectively). ( d ) Cumulative distributions of the OSIs determined for all responsive neurons recorded in APP23×PS45 mice at the different age groups ( n =95, 94, 149 and 145 neurons in 7, 6, 8 and 15 mice, respectively) as well as in 1.5–2-month-old and 8–10-month-old WT mice ( n =132 and 131 neurons in 7 and 13 mice, respectively). Functional impairments were observed only from the age of 4–4.5-months (Mann–Whitney test, APP23×PS45, 2-4-months, * P <0.005; 4–8-months, * P <0.005). ( e ) Proportion of highly (OSI>0.5) and broadly (OSI<0.5) tuned neurons in the visual cortex of APP23×PS45 mice (same neurons as in d ). Full size image We next investigated the visual performance of the APP23×PS45 mice and found that the aged (8- to 10-month-old) transgenic mice showed specific deficits in a visual pattern discrimination test [37] , [38] . ( Supplementary Methods ; Supplementary Fig. S3 ). Although the aged APP23×PS45 could discriminate drifting gratings of two orientations separated by 45°, they were not able to discriminate gratings that were just 22.5° apart, as indicated by the fact that their performance never exceeded the chance level ( Supplementary Fig. S3d , middle panel). It is important to note that young (3-month-old) APP23×PS45 mice, with only few plaques and relatively low levels of soluble Aβ present in their visual cortex ( Fig. 3b,c ), did not show such deficits in visual discrimination ( Supplementary Fig. S4 ). As a control, we performed an extra behavioural test to evaluate optomotor responses [39] ( Supplementary Fig. S5 ). It is known that optokinetic eye movements are largely driven by subcortical visual pathways [40] , [41] . We found that both aged WT and transgenic animals (8–10 months) had similar optomotor responses during the presentation of gratings ( Supplementary Fig. S5 ), indicating that the deficits observed in the visual discrimination task in the transgenic animals is not due to an alteration of retina function or of those subcortical pathways that are involved in optokinetic eye movements. In conclusion, the staged decline of neuronal function in the visual cortex of APP23×PS45 mice was associated with a decline in visual discrimination performance. Visually evoked versus spontaneous neuronal activity How does the impaired neuronal signalling in response to visual stimuli relate to the spontaneous activity? To address this question, we first performed a frequency analysis of the spontaneous activity in both WT and APP23×PS45 mice ( Fig. 4a,b ; Supplementary Fig. S6 ). We found that a substantial fraction of the neurons in the visual cortex of APP23×PS45 mice had activity patterns that were distinctly different from those encountered in the WT mice: some of the neurons displaying an increased activity (for example, Neuron 2, Fig. 4b ), while others being hypoactive or even silent (for example, Neuron 3, Fig. 4b ). In line with previous results obtained in the frontal cortex [26] , the neurons were classified based on their frequency of spontaneous calcium transients as 'normal' (frequency range: 0.25–4 transients per min), hypoactive (<0.25 transients per min) and hyperactive neurons (>4 transients per min) ( Supplementary Fig. S6a,b ). The analysis of the spontaneous activity clearly demonstrates that, in APP23×PS45 mice, the proportion of 'normal' neurons was substantially reduced, whereas the fraction of hypo- and hyperactive neurons was significantly larger ( Fig. 4c , Mann–Whitney test, hypoactive P <0.05, 'normal' P <0.001 and hyperactive neurons P <0.001). We determined the distribution of neurons as a function of their distance to the nearest plaque. The results show that there is a trend for hyperactive neurons to be more abundant near plaques ( Supplementary Fig. S7c ), although less pronounced than what had been reported for the frontal cortex [26] . Furthermore, in line with previous work, using a double transgenic model of AD [42] , we found an increase in the fraction of active astrocytes in the aged APP23×PS45 mice ( Supplementary Fig. S8b ). Notably, in parallel to the changes in Aβ-load and in neuronal orientation tuning ( Fig. 3 ), we found an age-dependent increase of both hypo- and hyper-active neurons (and a corresponding decrease in 'normal' neurons) ( Fig. 4d-f ). These results made us wonder whether the impaired tuning is a general feature of all neurons in APP23×PS45 mice, or whether impaired tuning is a particular problem of the hypo- or hyper-active neurons. 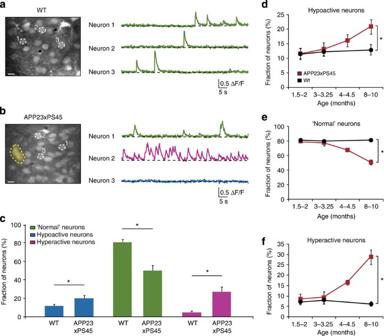Figure 4: Age-dependence of spontaneous activity in the visual cortex of WT and APP23×PS45 mice. (a,b) Spontaneous calcium transients recordedin vivofrom layer 2/3 neurons of the visual cortex of a WT (a) and an APP23×PS45 (b) mouse (10- and 9-months, respectively). Left panels,in vivotwo-photon images (z-stack, 0.5 μm step,±20 μm from the imaged focal plane). The broken yellow line delineates a Thioflavin-S positive plaque. Right panels, spontaneous calcium transients colour-coded according to the activity frequency: green for 'normal' neurons (0.25–4 transients per min), purple for hyperactive neurons (>4 transients per min) and blue for hypoactive neurons (0–0.25 transients per minute). Scale bar, 10 μm. (c) Bar graph showing the relative proportion of hypoactive, 'normal' and hyperactive neurons in 8–10-month-old WT and APP23×PS45 mice (n=630 and 806 neurons in 15 and 19 mice, respectively). Error bars indicate s.e.m. (Mann–Whitney test, hypoactive *P<0.05, 'normal' *P<0.001 and hyperactive neurons *P<0.001). (d–f) Proportion of hypoactive, 'normal' and hyperactive neurons in WT (black;n=686, 411, 630 neurons in 9, 5 and 15 mice, respectively) and APP23×PS45 (red;n=634, 620, 750 and 806 neurons in 10, 9, 10 and 19 APP23×PS45 mice, respectively) mice at four different age groups (1.5–2, 3–3.25, 4–4.5 and 8–10 months). Error bars indicate s.e.m. (Mann–Whitney test, hypoactive *P<0.05, 'normal' *P<0.001 and hyperactive neurons *P<0.001). Figure 4: Age-dependence of spontaneous activity in the visual cortex of WT and APP23×PS45 mice. ( a,b ) Spontaneous calcium transients recorded in vivo from layer 2/3 neurons of the visual cortex of a WT ( a ) and an APP23×PS45 ( b ) mouse (10- and 9-months, respectively). Left panels, in vivo two-photon images ( z -stack, 0.5 μm step,±20 μm from the imaged focal plane). The broken yellow line delineates a Thioflavin-S positive plaque. Right panels, spontaneous calcium transients colour-coded according to the activity frequency: green for 'normal' neurons (0.25–4 transients per min), purple for hyperactive neurons (>4 transients per min) and blue for hypoactive neurons (0–0.25 transients per minute). Scale bar, 10 μm. ( c ) Bar graph showing the relative proportion of hypoactive, 'normal' and hyperactive neurons in 8–10-month-old WT and APP23×PS45 mice ( n =630 and 806 neurons in 15 and 19 mice, respectively). Error bars indicate s.e.m. (Mann–Whitney test, hypoactive * P <0.05, 'normal' * P <0.001 and hyperactive neurons * P <0.001). ( d–f ) Proportion of hypoactive, 'normal' and hyperactive neurons in WT (black; n =686, 411, 630 neurons in 9, 5 and 15 mice, respectively) and APP23×PS45 (red; n =634, 620, 750 and 806 neurons in 10, 9, 10 and 19 APP23×PS45 mice, respectively) mice at four different age groups (1.5–2, 3–3.25, 4–4.5 and 8–10 months). Error bars indicate s.e.m. (Mann–Whitney test, hypoactive * P <0.05, 'normal' * P <0.001 and hyperactive neurons * P <0.001). Full size image To deal with this question, we initially determined the activity status ('normal', hypo- or hyper-active) of the neurons in the field of view by recording their spontaneous activity during at least 4 min, and we then imaged their activity evoked by drifting gratings of different orientations. We first focused on the neurons that had a 'normal' frequency of their spontaneous activity. Fig. 5a illustrates the results obtained from such a 'normal' neuron. We found that this neuron responded specifically to one orientation of drifting gratings, but not to all the other directions. For this neuron, we calculated an OSI of 0.99 and a DSI of 0.47, values that were strikingly similar to highly tuned neurons in WT mice ( Fig. 5b ; see also Fig 1c ). The overlaid polar plots of large numbers of 'normal' neurons of both genotypes (WT, n =107 and APP23×PS45, n =67 neurons) and the calculated median tuning functions revealed a high degree of similarity ( Fig. 5c ). Accordingly, the cumulative distributions of OSIs and DSIs did not show any significant difference in the two genotypes ( Fig. 5d , Mann–Whitney test, OSI, P =0.39; DSI, P =0.92). Furthermore, the amplitudes of spontaneous and visually evoked calcium transients were also similar in both genotypes ( Supplementary Fig. S9b ). These results strongly indicate that, in APP23×PS45 mice, the fraction of neurons, with a 'normal' spontaneous activity, has tuning properties, for both orientation and direction, which are indistinguishable from those found in WT mice. 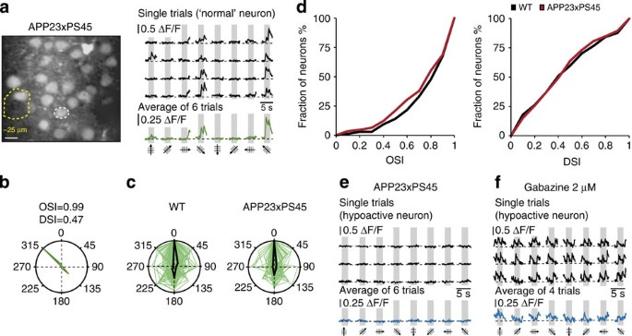Figure 5: Response of normal and hypoactive neurons to stimulus orientation and direction. (a) Left panel,in vivotwo-photon image of layer 2/3 neurons in the visual cortex of an APP23×PS45 mouse (8-months). The broken yellow line delineates a Thioflavin-S-positive plaque that was located 25 μm below the imaged focal plane (seen on thez-stack). Right panel, calcium transients evoked by visual stimulation in the 'normal' neuron indicated in the left panel by a white-dotted circle. Scale bar, 10 μm. (b) Polar plot showing the neuron's response function to oriented drifting gratings. The responses to each of the eight directions tested were normalized with respect to the maximal response. Then, the function was constructed by connecting the eight values. (c) Overlap of the polar plots obtained for all responsive 'normal' neurons recorded in 13 WT (n=107 neurons) and 15 APP23×PS45 (n=67 neurons) mice. Polar plots were normalized to a preferred direction of 0° and maximal response. Black lines indicate median tuning function. (d) Cumulative distributions of the orientation (OSI) and direction (DSI) selectivity indices determined for all 'normal' neurons recorded in 13 WT (black) and 15 APP23×PS45 (red) mice. 'Normal' neurons were similarly tuned for orientation and direction in both APP23×PS45 and WT mice (Mann–Whitney test, OSI,P=0.39; DSI,P=0.92). (e) Calcium imaging of a hypoactive neuron's activity recorded during visual stimulation in the layer 2/3 of an APP23×PS45 mouse (8.5-months). Four single trials are represented with black lines and the average of six trials is shown in blue. (f) Calcium transients recorded from the same neuron as in paneleafter application of gabazine. Figure 5: Response of normal and hypoactive neurons to stimulus orientation and direction. ( a ) Left panel, in vivo two-photon image of layer 2/3 neurons in the visual cortex of an APP23×PS45 mouse (8-months). The broken yellow line delineates a Thioflavin-S-positive plaque that was located 25 μm below the imaged focal plane (seen on the z -stack). Right panel, calcium transients evoked by visual stimulation in the 'normal' neuron indicated in the left panel by a white-dotted circle. Scale bar, 10 μm. ( b ) Polar plot showing the neuron's response function to oriented drifting gratings. The responses to each of the eight directions tested were normalized with respect to the maximal response. Then, the function was constructed by connecting the eight values. ( c ) Overlap of the polar plots obtained for all responsive 'normal' neurons recorded in 13 WT ( n =107 neurons) and 15 APP23×PS45 ( n =67 neurons) mice. Polar plots were normalized to a preferred direction of 0° and maximal response. Black lines indicate median tuning function. ( d ) Cumulative distributions of the orientation (OSI) and direction (DSI) selectivity indices determined for all 'normal' neurons recorded in 13 WT (black) and 15 APP23×PS45 (red) mice. 'Normal' neurons were similarly tuned for orientation and direction in both APP23×PS45 and WT mice (Mann–Whitney test, OSI, P =0.39; DSI, P =0.92). ( e ) Calcium imaging of a hypoactive neuron's activity recorded during visual stimulation in the layer 2/3 of an APP23×PS45 mouse (8.5-months). Four single trials are represented with black lines and the average of six trials is shown in blue. ( f ) Calcium transients recorded from the same neuron as in panel e after application of gabazine. Full size image In contrast to the 'normal' neurons, the fraction of hypoactive neurons, which included both the totally silent neurons and the neurons with a very low frequency of spontaneous activity (<0.25 transients per min), were characterized by a total absence of visually evoked responses ( Fig. 5e ). A similar complete absence of visually evoked responses was observed in all hypoactive neurons tested ( n =90 neurons in 15 mice) in APP23×PS45 mice. It is interesting to note that, in WT animals, 20% of the hypoactive neurons (11 out of 55 neurons tested in 13 mice) did respond normally to visual stimulation with drifting gratings and, in fact, had tuning properties for orientation and direction that were similar to those obtained for 'normal' neurons (Mann–Whitney test, OSI, P =0.67; DSI P =0.17). These observations suggest that there is a difference between hypoactive neurons of WT and APP23×PS45 mice. One possibility is that hypoactive neurons in the visual cortex of APP23×PS45 mice are unable to fire, because they have impaired membrane properties. Alternatively, they can still fire action potentials, but they are silenced by inhibitory inputs. To address this issue, we applied the GABA A receptor antagonist gabazine and found that spontaneous activity could be restored with this treatment ( Supplementary Fig. S7a,b ). However, except for random calcium transients during single-trial recordings, no clear and reliable visually evoked responses were resolved in the disinhibited neurons ( Fig. 5f ). Thus, hypoactive neurons preserve some functional intrinsic properties, but seem to lack the mechanisms responsible for the detection of sensory-evoked signals. Impaired tuning of hyperactive neurons of APP23×PS45 mice In a next attempt to identify the poorly tuned neurons that are frequently encountered in the diseased cortex, we focused on the hyperactive neurons. Fig. 6a shows the stimulus-evoked responses of a hyperactive neuron. This neuron was poorly tuned and produced large calcium transients in response to several orientations and directions (6/8) of the drifting gratings ( Fig. 6b top panel, OSI=0.38, DSI=0.07). Similar broad tuning levels were found to be a general property of all the hyperactive neurons in aged APP23×PS45 mice ( Fig. 6b , lower panel). This conclusion is strikingly illustrated by the comparison of the cumulative distributions of the OSIs of hyperactive and 'normal' neurons in APP23×PS45 mice, showing the age dependence of hyperactive neurons impairment ( Supplementary Fig. S9a , 4–4.5 months, Mann–Whitney test, P <0.001; 8–10 months, Mann–Whitney test, OSI, P <0.001). 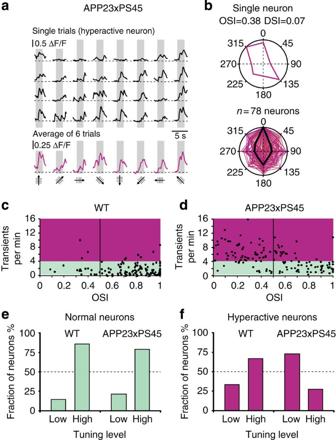Figure 6: Response of hyperactive neurons to stimulus orientation and direction. (a) Stimulus-evoked calcium transients recorded from a hyperactive neuron in an APP23×PS45 mouse (8-months). (b) Top panel, polar plot showing the response function (purple lines) to oriented drifting gratings of the same neuron as in panela. Lower panel, overlap of the polar plots obtained for all responsive hyperactive neurons recorded in 15 APP23×PS45 mice (n=78 neurons). Polar plots were normalized to a preferred direction of 0° and maximal response. Black lines indicate median tuning function. (c,d) Scatter plots showing the relation between the OSI and the frequency of spontaneous calcium transients in WT (c) and APP23×PS45 (d) mice (n=131 and 145 neurons from 13 and 15 mice, respectively). The coloured areas indicate the frequency domains of 'normal' (green) and hyperactive (purple) spontaneous activity. (e,f) Comparison of the fractions of 'normal' (e) and hyperactive (f) neurons with low (OSI<0.5) and high orientation tuning (OSI>0.5) levels in WT and APP23×PS45 mice (same neurons as inc,d). Figure 6: Response of hyperactive neurons to stimulus orientation and direction. ( a ) Stimulus-evoked calcium transients recorded from a hyperactive neuron in an APP23×PS45 mouse (8-months). ( b ) Top panel, polar plot showing the response function (purple lines) to oriented drifting gratings of the same neuron as in panel a . Lower panel, overlap of the polar plots obtained for all responsive hyperactive neurons recorded in 15 APP23×PS45 mice ( n =78 neurons). Polar plots were normalized to a preferred direction of 0° and maximal response. Black lines indicate median tuning function. ( c,d ) Scatter plots showing the relation between the OSI and the frequency of spontaneous calcium transients in WT ( c ) and APP23×PS45 ( d ) mice ( n =131 and 145 neurons from 13 and 15 mice, respectively). The coloured areas indicate the frequency domains of 'normal' (green) and hyperactive (purple) spontaneous activity. ( e,f ) Comparison of the fractions of 'normal' ( e ) and hyperactive ( f ) neurons with low (OSI<0.5) and high orientation tuning (OSI>0.5) levels in WT and APP23×PS45 mice (same neurons as in c,d ). Full size image In view of the impaired tuning of hyperactive neurons, it is interesting to ask whether the frequency of spontaneous activity correlates inversely with the tuning performance over the entire frequency range. In WT mice, there was no evidence for such a correlation and a high OSI was determined for the majority of both normal and hyperactive neurons, as indicated by the scatterplot shown in Fig. 6c . By contrast, the results obtained for APP23×PS45 mice showed that the vast majority of neurons with a low OSI were in the upper-left quadrant of the scatter plot, whereas the neurons with a high OSI were in the lower-right quadrant, corresponding to the 'normal' frequency range ( Fig. 6d ). A quantitative comparison for the two genotypes underscored this impression by showing that the proportion of 'normal' neurons with high-and-low OSI values was similar ( Fig. 6e ). Instead, there was a striking contrast between the hyperactive neurons in the two genotypes ( Fig. 6f ). Whereas the hyperactive neurons of WT mice had mostly a high OSI, the hyperactive neurons of APP23×PS45 mice had mostly low OSI values. This indicates that high spontaneous activity per se does not explain the loss in orientation tuning. To verify this conclusion independently, we analysed periods of spontaneous activity by randomly assigning periods of nominal stimulation (see Methods ). The results demonstrate that even in conditions of high spontaneous activity, the level of false positive responses is low ( Supplementary Fig. S10 ). Together, these results establish that a major source for the impaired orientation and direction tuning in APP23×PS45 mice is the hyperactive neurons and that this loss of tuning is not due to a simple increase in spontaneous activity, but to qualitative functional changes that are disease specific. In this study, we obtained direct insights into the relation between the age-dependent increase of Aβ-load, specific changes in the function of cortical neurons in vivo and behavioural alterations in a mouse model of AD. First, we found that the staged increase of Aβ-load, including both insoluble Aβ-plaques and soluble Aβ, in the visual cortex, was paralleled by reduced orientation and direction tunings of many neurons as well as reduced performance in a visual discrimination test. Second, the spontaneous ongoing activity of a large fraction of neurons was also massively changed in the visual cortex of APP23×PS45 mice, with substantial fractions of hypo- and hyper-active neurons. Third, while hypoactive neurons were entirely unresponsive to visual stimuli, we found that impaired orientation and direction tuning was primarily due to massively impaired performance of the hyperactive neurons. Together, the results establish that there is a parallel progression in the change of Aβ-load, cortical dysfunction and sensory deficits in the APP23×PS45 mouse model of AD. In vivo two-photon imaging in animal models advanced substantially our understanding of the pathomechanisms that underlie AD [20] , [21] , [31] , [43] . Several studies have analysed the morphological and activity changes of neurons. They revealed neuritic dystrophies and a loss of dendritic spines [20] , [43] , an increased resting calcium level in a subset of dendrites [21] , an increase in activity and resting calcium concentration in glial cells [42] , as well as an increase in the fraction of hyperactive neurons [26] . In this study, we used in vivo two-photon calcium imaging to analyse sensory-evoked neuronal signals in the APP23×PS45 mouse model. We found in this mouse model an age-dependent increase of Aβ in the visual cortex. Furthermore, in the diseased visual cortex of these mice, the orientation and direction tuning of many neurons was substantially lower than in WT mice. It is important to note that in the young transgenic mice, in which Aβ-aggregates were absent, the tuning level of the neurons was not different from that of WT mice of the same age. This is an indication that visual cortex development of APP23×PS45 transgenic mice, during the first postnatal months, is not disrupted. The overview of the age-related changes illustrated in Table 1 suggests that the decline in visual processing can be associated with distinct stages [6] . In our mouse model of AD, stage I lasts from birth until the age of about 3 months. During this early period, visual discrimination and visual cortex function are normal, while plaques are largely absent and soluble Aβ-levels are moderately increased. The results obtained in 4–4.5-month-old mice revealed an intermediate stage, stage II, in which the plaques were present at substantial higher densities in the visual cortex, soluble Aβ-levels were also higher and orientation/direction tuning of visual cortex neurons showed significant signs of impairment. Finally, the most severe changes were found at the age of 7–8 months, corresponding to stage III. At stage III, all parameters tested, namely, plaque density, soluble Aβ-concentration, orientation tuning and visual discrimination deviated most severely from the control values obtained in WT mice. It is important to note that, while nearly 50% of the neurons in the primary visual cortex were functionally impaired, the transgenic mice were still able to discriminate gratings differing by 45°. This indicates that even a reduced circuit of 'normal' neurons is largely capable of sustaining physiological activities, perhaps with the help of compensatory mechanisms [23] , [44] . Such reduced circuits may account for the observations in humans that apparently normal cognitive function is largely sustained, despite the presence of substantial neuropathology in their brains [45] , [46] . Table 1 Staged decline of visual processing in the APP23×PS45 mouse model. Full size table The mechanisms underlying the changed neuronal activity in the diseased visual cortex are likely to involve a redistribution of synaptic inhibition [47] and excitation [24] , as it has been proposed for the impaired spontaneous activity in the frontal cortex [26] . This is suggested by the observation that similar fractions of hypo- and hyper-active neurons were detected in both cortical regions. Furthermore, application of the GABA A receptor antagonist gabazine was able to induce neuronal activity in hypoactive neurons, indicating that excessive inhibition is one of the reasons for the impaired network activity. Interestingly, chronic functional impairments, by traumatic or ischemic lesions of the cortex, share important similarities with those observed in the Aβ-containing cortical regions, which are enriched with hyperactive neurons. For example, it is clinically well established that the cortical area that is adjacent to the traumatically destroyed cortical tissue is a trigger site for post-traumatic epileptic seizures [48] . Furthermore, a strong increase of neuronal excitability has been observed in regions surrounding experimental cortical lesions in the cat visual cortex [49] . This hyperexcitability was shown to cause an increase in both spontaneous and visually evoked activity. The major consequence of the functional reorganization in the cortical region surrounding the lesion was the enlargement of receptive fields that included the lost parts of the visual field representation [50] , [51] . It was suggested that neurons at the border of a lesion receive subthreshold inputs outside their original receptive field and that these inputs become functional after the lesion [50] , [51] . Finally, in rodent models of stroke, post-lesion hyperexcitability was shown to develop in the somatosensory cortex over the first week to month after the incident [52] , [53] . In addition, an expansion of the receptive field size and a loss of specificity in the neuron's response to sensory stimulation were found in the peri-infarct region [52] . In vivo two-photon calcium imaging showed that the limb selectivity of individual neurons was altered after the stroke such that neurons that were previously selective for a single contralateral limb processed information from multiple limbs [52] . In analogy to these findings, Aβ-plaques can be interpreted as multiple small cortical lesions, causing hyperexcitability and loss of functional selectivity owing to structural and functional changes in their vicinity. In addition, soluble Aβ may form a synaptotoxic microenvironment for the neurons surrounding the Aβ-plaques [31] . The precise cellular mechanisms underlying the hyperexcitability in AD will need to be established in future studies. Some mechanisms may be similar to those suggested to contribute to the hyperactivity observed after brain injuries that cause post-traumatic epilepsy. They include sprouting of excitatory inputs, loss of GABAergic inhibition and loss of trophic support normally provided by brain-derived neurotrophic factor (for review, see ref. 54 ). Animals and surgery All experimental procedures were performed in accordance with institutional animal welfare guidelines and were approved by the Government of Bavaria, Germany. APP23×PS45 mice were generated from two already existing transgenic mouse lines as described previously [26] . Briefly, one line, APP23 [32] , overexpresses human amyloid precursor protein (APP) with the Swedish double mutation at positions 670/671, whereas the other, PS45 (ref. 33 ) carries a transgene for the human Presenilin 1 bearing the G384A mutation (both lines are driven by a Thy-1 promoter). APP23×PS45 mice were reared in 12/12 h light/dark cycles (P46-P60, n =10; 3–3.25 months, n =9; 4–4.5 months, n =10; 8–10 months, n =19). These mice were compared with WT mice with the same strain background (C57Bl/6) and of similar ages (P55-P60, n =9; 3–3.25 months, n =5; 8–10 months, n =15) and to the PS45 mouse line (8–10 months, n =5). Genotypes were systematically determined by PCR analysis. Animals were prepared for in vivo two-photon calcium imaging, as described previously [29] . Briefly, the mice were placed onto a warming plate (38 °C) and anaesthetized by inhalation of 1.5% isoflurane (Curamed, Karlsruhe, Germany) in pure O 2 . After removing the skin, a custom-made recording chamber [55] was then glued to the skull with cyanoacrylic glue (UHU, Buhl-Baden, Germany). The mouse was then transferred into the set-up, placed onto a warming plate (38 °C), and continuously supplied with 0.8–1% isoflurane in pure O 2 (breathing rate, 110–130 b.p.m.). The position of the primary visual cortex was located according to brain atlas coordinates (Bregma −3 to −4.5, 2–3 mm lateral to the midline) [56] . In all experiments, the correct location of the imaged neurons was confirmed post-hoc by imaging of the stained brain area (for example, Fig. 1a ). A small craniotomy (~0.8×0.6 mm) was performed above the monocular region of primary visual cortex using a thin (30-gauge) injection needle. The recording chamber was perfused with warm (37 °C) extracellular perfusion saline containing (in mM): 125 NaCl, 4.5 KCl, 26 NaHCO 3 , 1.25 NaH 2 PO 4 , 2 CaCl 2 , 1 MgCl 2 , 20 glucose, pH 7.4, when bubbled with 95% O 2 and 5% CO 2 . The neurons were stained in vivo with the fluorescent calcium indicator dye Oregon Green BAPTA-1 (OGB-1) following the protocol described in detail in ref. 29 . Amyloid-β-plaques were stained in vivo in a comparable way, by pressure-injecting Thioflavin-S (0.001% (w/v)). Eye cream (Bepanthen, Bayer) was applied on both eyes to prevent dehydration during surgery. After surgery, the anaesthesia level was decreased to 0.8% isoflurane for recordings (breathing rate, 110–130 b.p.m.). Two-photon calcium imaging In vivo calcium imaging was performed by using a custom-built two-photon microscope based on Ti:Sapphire pulsing laser (model: Chameleon, repetition rate: 80 MHz, pulse width: 140 fs; Coherent) and resonant galvo-mirror (8 kHz; GSI) system [57] . The scanner was mounted on an upright microscope (BX51WI, Olympus, Tokyo, Japan) equipped with a water-immersion objective (×60, 1.0 NA Nikon, Japan or ×40, 0.8″ NA Nikon, Japan). Emitted photons were detected by photomultiplier tubes (H7422-40; Hamamatsu). Full-frame images at 480×400 pixel resolution were acquired at 30 Hz by custom-programmed software based on LabVIEW (version 8.2; National Instruments). At each focal plane, we imaged spontaneous activity (for at least 4 min) as well as visually evoked activity (6 to 10 trials of visual stimulation). For simultaneous visualization of Aβ-plaques and cortical neurons labelled with OGB-1, the emitted fluorescence light was split at 515 nm. To identify the amyloid plaques close to the recorded neurons, the brain region (± about 200 μm, centred on the recorded neurons) was scanned through in the z direction (z-stack, 2 μm step), at the end of each experiment. Drug application Gabazine (2 μM) was added to the extracellular saline solution perfusing the chamber attached to the mouse's skull ('bath' application). Visual stimulation Visual stimuli were generated by Matlab (release 2007b; Mathworks) with the 'Psychtoolbox' add-on package ( http://psychtoolbox.org/wikka.php?wakka=HomePage ). Visual stimuli were projected on a screen placed 30 cm from the contralateral eye, covering 80°×67° of the visual field. Each trial of visual stimulation started with a grey screen (mean luminance) for 5 s, followed by a stationary square-wave grating for 4 s and the corresponding drifting phase for 2 s (0.03 c.p.d., 1 Hz, 8 directions, contrast 80%, mean luminance 3.7 cd m −2 ). We used stationary gratings during the inter-stimulus periods to study specifically the responses to moving gratings. When a blank screen is used during the inter-stimulus period instead of stationary gratings, responses to local changes in luminance may occur. At each focal plane, evoked activities were imaged during 6–10 trials. Under our experimental conditions, this visual stimulation protocol evoked visual responses in 95/313 neurons (APP23×PS45, 1.5–2 months), 132/426 neurons (WT, 1.5–2 months), 94/334 neurons (APP23×PS45, 3–3.25 months), 140/464 neurons (APP23×PS45, 4–4.5 months), 145/404 neurons (APP23×PS45, 8–10 months) and in 131/384 neurons (WT, 8–10 months). Data analysis The image analysis was performed off-line in two steps. First, the ImageJ software (http://rsb.info.nih.gov/ij/) was used for drawing regions of interest (ROIs) around cell bodies and around a large area of cell-free neuropil. Astrocytes were identified based on their selective staining by sulforhodamine 101 (refs 58 , 59 ), brighter appearance after staining with OGB1-AM 35 and their specific morphology with clearly visible processes. The presence of glial processes was assessed by inspecting 3D-stacks (70 μm below and upper the imaged plane) obtained routinely at the end of each experiment. In the next step, custom-made routines of the Igor Pro software (Wavemetrics, Lake Oswego, Oregon, USA) were used for the detection of wave-associated calcium transients in individual neurons. Calcium signals were expressed as relative fluorescence changes (ΔF/F) corresponding to the mean fluorescence from all pixels within specified ROIs. For each ROI, a transient was accepted as a signal, when its peak amplitude was greater than three times the standard deviation of the noise band. After the automatic analysis, all traces were carefully inspected. The analysis of the visually evoked responses was performed by using the average traces of the 6–10 stimulus trials used during the imaging session (see examples in Figs 1,2 1b and 2b). Neurons were defined as responsive to moving gratings when they responded to at least one of the eight directions with a significant change in fluorescence (mean amplitude during the 2 s of stimulus presentation, t-test) compared with the activity during the 2 s preceding the presentation of the stimulus (standing grating). An OSI (for example, ref. 36 ) was calculated to quantify the tuning level of the neurons with regard to the orientation of the drifting grating. The OSI was defined as ( R pref − R ortho )/( R pref + R ortho ), where R pref , the mean response in the preferred orientation, was the response with the largest magnitude in the average trace of the 6–10 trials. R pref was determined as the mean of the integrals of the calcium transients for the two corresponding opposite directions. R ortho was similarly calculated as the response evoked by the orthogonal orientation. With this index, perfect orientation selectivity would give OSI=1; an equal response to all orientations would have OSI=0, and 3:1 selectivity corresponds to OSI=0.5. Highly and poorly tuned neurons were defined as neurons with an OSI>0.5 and OSI<0.5, respectively. Similarly, a DSI was defined as (R pref −R opp )/(R pref +R opp ), where R opp is the response in the direction opposite to the preferred direction. Polar plots show neuron response function to oriented drifting gratings. The mean responses to each of the eight directions tested were normalized with respect to the maximal response. Then, the function was constructed by connecting the eight values. Statistical analysis The following values were compared between APP23×PS45 and WT mice using a Mann–Whitney test with a two-tailed level of significance set at α =0.05. (SPSS 16.0 software): fraction of 'normal', hypoactive and hyperactive neurons, cumulative distributions of OSI and DSI, and percentages of good choices in the pattern discrimination task. The last values were also compared with chance level using a nonparametric χ 2 test. Measurement of plaque load in situ Coronal brain slices were obtained from brains imaged in vivo. After fixation with 4% paraformaldehyde, 25 μm-cryosections of the visual cortex were prepared. Sections were washed in PBS, before heat-induced antigen retrieval (90 °C for 5 min) in 0.1 M citric acid buffer. For the detection of Aβ-deposition, two different methods were applied: immunohistological staining with the 4G8 antibody and Thioflavin-S staining. For the first one, we used primary mouse anti-human Aβ-antibody 4G8 (Covance, Princeton, NJ, USA) with a dilution of 1:1,000 and a secondary biotinylated horse anti-mouse IgG antibody (BA2000, Vector Laboratories, Burlingame, CA, USA) diluted 1:200. The slices were further processed using the Vectorstain Elite ABC Kits (Vector). After the reaction with Diaminobenzidine (Roche, Code 17118096), the slices were dehydrated and cover slipped. Thioflavin-S (0.05% (w/v) in 50% ethanol) was applied for 8 min in darkness by bath application. This was followed by two differentiation steps in 80% ethanol for 10 s each, three washes in distilled water and 30-min washout of the residual dye in a concentrated phosphate buffer [60] . Micrographs were taken using a camera (XC10, Olympus, Tokyo, Japan) mounted on an Olympus microscope (MVX10, Olympus, Tokyo, Japan). The images were processed offline using the ImageJ program ( http://rsb.info.nih.gov/ij/ ). To determine the plaque density, PFA-fixed slices (200-μm thick) were stained by bath application of Thioflavin (0.005% (w/v)) for 20 min. After 20 min, washout of the residual dye images were taken and processed as described above. The plaque density (in per cent) was then calculated as the relative fraction of green pixels. Determination of amyloid-β Frozen forebrain hemispheres (excluding hindbrain and olfactory bulb) from the four different age groups (1.5–2, 3–3.25, 4–4.5 and 8–10 months) were weighed and homogenized at 10% (w/v) in Tris-buffered saline (30 mM Tris–HCl pH 7.6, 137 mM sodium chloride, protease inhibitor cocktail cOmplete, Roche Molecular Biochemicals), using Eppendorf micropestles (Vaudaux-Eppendorf, Schönenbuch, Basel, Switzerland). Aliquots for the analysis of soluble Aβ were removed and stored at -80° until analysis. Quantitative determinations of Aβ were done with electrochemoluminescence-linked immunoassays (Human Aβ40 and Aβ42 Ultrasensitive Kits, Meso Scale Discovery, Gaithersburg, MD). Standard curves with synthetic Aβ1–40 (Bachem) and 1–42 (rPeptide) were set up in non-transgenic mouse forebrain extract, prepared identically to the transgenic samples. For analysis of soluble Aβ, 50 μl of each forebrain homogenate were supplemented with 1 volume of Tris-buffered saline and extracted for 15 min at 4 °C. Homogenates were mixed every 5 minutes. The supernatants of a 15-min centrifugation at 100,000 g were diluted with 9 volumes of blocking solution from the immunoassay kit. 25 μl of each sample were loaded as duplicates on the assay plates and further processed, according to the manufacturer's protocol. For quantification of total Aβ, homogenates were sonicated on ice, supplemented with concentrated formic acid (final concentration 70%) and extracted for 15 min at 4 °C, with occasional mixing. Extracts were neutralized by addition of 19 volumes 1 M Tris and centrifuged at 20,000 g for 15 min at 4 °C. The supernatants were either diluted with 6.5 volumes (2–3 months-old animals), or with 149 volumes (4–8 months-old animals) of blocking solution from the immunoassay kit. Aβ-concentrations were read from the standard curves using a point-to-point fit with the software Softmax Pro 4.0 (Molecular Devices, Sunnyvale, CA, USA). How to cite this article: Grienberger, C. et al . Staged decline of neuronal function in vivo in an animal model of Alzheimer's disease. Nat. Commun. 3:774 doi: 10.1038/ncomms1783 (2012).